Theoretical prediction of a strongly correlated Dirac metal Recently, the most intensely studied objects in the electronic theory of solids have been strongly correlated systems and graphene. However, the fact that the Dirac bands in graphene are made up of sp 2 electrons, which are subject to neither strong Hubbard repulsion U nor strong Hund’s rule coupling J , creates certain limitations in terms of novel, interaction-induced physics that could be derived from Dirac points. Here we propose GaCu 3 (OH) 6 Cl 2 (Ga-substituted herbertsmithite) as a correlated Dirac–Kagome metal combining Dirac electrons, strong interactions and frustrated magnetic interactions. Using density functional theory, we calculate its crystallographic and electronic properties, and observe that it has symmetry-protected Dirac points at the Fermi level. Its many-body physics is diverse, with possible charge, magnetic and superconducting instabilities. Through a combination of various many-body methods we study possible symmetry-lowering phase transitions such as Mott-Hubbard, charge or magnetic ordering, and unconventional superconductivity, which in this compound assumes an f -wave symmetry. It is well known theoretically that graphene is not the only system in which crystallography, combined with a particular one-electron Hamiltonian, creates symmetry-protected Dirac points at a certain filling. As such, hope persists to combine the features of Dirac fermions and strong correlations in an experimentally accessible condensed matter system. For instance, the single-orbital kagome tight-binding model is known to feature, besides a flat band that has been a subject of considerable interest, symmetry-protected Dirac points at a filling of n =4/3 electrons per site (or, equivalently, 1/3, for the reversed sign of the hopping). However, so far this fact has been considered more a numerical curiosity of a simplified model than an accessible feature in real materials, and has received little attention. Currently, the predominantly studied kagome material has been herbertsmithite [1] , [2] , [3] , ZnCu 3 (OH) 6 Cl 2 , presumed to host a spin liquid with fractionalized spin excitations, consistent with recent neutron-scattering measurements [4] . It might be the first manifestation of a truly two-dimensional resonating valence bond (RVB) spin liquid anticipated 41 years ago [5] and intensively discussed in the framework of high-temperature superconductivity in cuprates [6] , [7] , [8] , [9] . The possibility of an RVB spin liquid in the kagome lattice is presently supported by large-scale numerical investigations [10] , [11] , [12] , [13] . Herbertsmithite [14] is the starting point of our proposal to unify strong correlations, metallicity and Dirac fermions. As opposed to the flat band that only exists in the nearest-neighbour single-orbital tight-binding model, the Dirac points in the kagome compounds are symmetry protected and survive in any electronic structure model that respects the hexagonal symmetry. By replacing Zn 2+ with Ga 3+ in herbertsmithite, GaCu 3 (OH) 6 Cl 2 ( Fig. 1 ), the Dirac points are placed at the Fermi level. These states are formed by the strongly correlated ( U / t ~20) orbitals, whose nearest-neighbour hopping Hamiltonian on the kagome lattice, after integrating out the oxygens, appears to be equivalent to that of directly overlapping s orbitals. As we will further elaborate on below, compared to graphene, we find a strong screening, hinting at rather local interactions, while the nature of magnetic interactions is typical for the kagome lattice, suggesting no long-range antiferromagnetism and a dispersionless spin fluctuation profile. 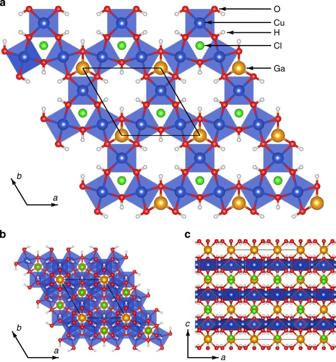Figure 1: Structure of predicted herbertsmithite modification GaCu3(OH)6Cl2. (a) View of an individual kagome plane. (b) Full view alongcaxis where three shifted kagome layers are stacked. (c) Side view. Figure 1: Structure of predicted herbertsmithite modification GaCu 3 (OH) 6 Cl 2 . ( a ) View of an individual kagome plane. ( b ) Full view along c axis where three shifted kagome layers are stacked. ( c ) Side view. Full size image Zn and Ga are neighbours in the periodic table and their radii are similar. Even if they do not form a continuous solid solution, our calculations suggest that the fully substituted compound, GaCu 3 (OH) 6 Cl 2 , should be dynamically stable, and it should be possible to dope it with holes by partially replacing Ga with Zn. If the solid solution Zn 1− x Ga x Cu 3 (OH) 6 Cl 2 were to exist, it would span the whole range from a fully frustrated RVB spin liquid ( x =0) at half filling ( n =1) to a strongly correlated Dirac metal ( x =1) at n =4/3. The ground state in the former limit is known to be a uniform Mott insulator. Upon doping, a number of instabilities can manifest themselves, and in fact one can anticipate a complex and highly interesting phase diagram. Specifically, the density functional theory (DFT) noninteracting one-electron picture may be prone to Mott–Hubbard metal–insulator transition, charge ordering, ferromagnetism or a superconducting instability. Below we will first present our DFT calculations, and then discuss these possible instabilities by means of various complementary many-body model approaches. First-principles calculations Herbertsmithite is part of the Zn-paratacamite family of compounds [3] that shows great flexibility in its composition both naturally (for example, Ni-herbertsmithite [15] ) and synthetically (for example, Mg-herbertsmithite [16] ). Substitution of Zn 2+ by Ga 3+ poses a bigger challenge for solid-state chemists due to the different oxidation and the fact that Ga more commonly assumes a fourfold coordination. Nevertheless, it has been shown that the sixfold coordination is also possible [17] . In the framework of DFT we fully relaxed the herbertsmithite structure after replacing Zn by Ga (see Supplementary Note 1 ). The resulting electronic structure ( Fig. 2c ) shows low-energy bands qualitatively similar to a one-orbital model on the kagome lattice ( Fig. 2a ) and has Dirac points exactly at the Fermi level. In order to understand this fact, we first observe that Cu in this structure sits inside an oxygen square, so that the orbitals, with strong pdσ hopping t pdσ to the oxygens, form a high-lying antibonding band ( Fig. 3 ). If one neglects the other d orbitals, and integrates out oxygens, one gets a tight-binding model, which is mathematically equivalent to a single s -orbital model with the nearest-neighbour hopping where E d and E p are the energies of the d and p orbitals, respectively. The solution of this model is well known ( Fig. 2a ). The bands crossing along the Γ− K line have different parity with respect to the y /− y transformation ( y ⊥ Γ K ), and therefore the Dirac points at K are symmetry-protected for an arbitrary hopping range (apart from the very small spin–orbit coupling). 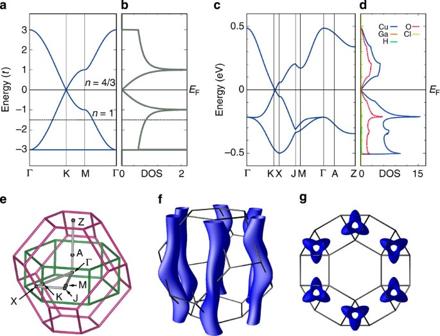Figure 2: Electronic structure of GaCu3(OH)6Cl2. (a) Band structure and (b) density of states of the nearest-neighbour tight-binding model for the kagome lattice. (c–g) Electronic structure of Ga-substituted herbertsmithite, GaCu3(OH)6Cl2. (c) Band structure along high symmetry points of the hexagonal setting of thespace group. (d) Density of states showing GaCu3(OH)6Cl2to be a zero-gap semiconductor. (e) Brillouin zones of thespace group in rhombohedral (purple) and hexagonal setting (green), with the path chosen inc(see also a view from the top inSupplementary Fig. 1). (f,g) Fermi surfaces at an energyE=−60 meV. The Fermi surface plots demonstrate that the material is two-dimensional to a good approximation. Figure 2: Electronic structure of GaCu 3 (OH) 6 Cl 2 . ( a ) Band structure and ( b ) density of states of the nearest-neighbour tight-binding model for the kagome lattice. ( c – g ) Electronic structure of Ga-substituted herbertsmithite, GaCu 3 (OH) 6 Cl 2 . ( c ) Band structure along high symmetry points of the hexagonal setting of the space group. ( d ) Density of states showing GaCu 3 (OH) 6 Cl 2 to be a zero-gap semiconductor. ( e ) Brillouin zones of the space group in rhombohedral (purple) and hexagonal setting (green), with the path chosen in c (see also a view from the top in Supplementary Fig. 1 ). ( f , g ) Fermi surfaces at an energy E =−60 meV. The Fermi surface plots demonstrate that the material is two-dimensional to a good approximation. 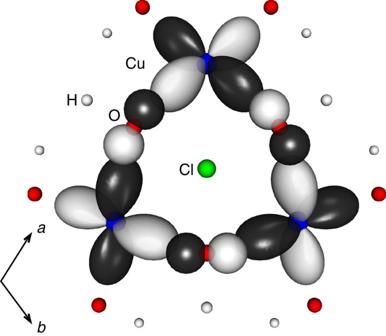Figure 3: Relevant tight-binding orbitals for GaCu3(OH)6Cl2. Overlap between Cuand Oporbitals in a Cu triangle. + and − signs of the wave function are coded with black and white, respectively. Full size image Figure 3: Relevant tight-binding orbitals for GaCu 3 (OH) 6 Cl 2 . Overlap between Cu and O p orbitals in a Cu triangle. + and − signs of the wave function are coded with black and white, respectively. Full size image The kagome tight-binding model has Dirac points at K ; however, this is not the case for a finite k z dispersion and rhombohedral symmetry ( Fig. 2c ). In a planar system with hexagonal symmetry one can travel from Γ to M and then continue to another Γ. In a rhombohedral structure, if one travels along the same direction one actually ends up at Z , and the k z =0 plane alone has lower symmetry than if averaged over all k z . The Dirac points are not anymore located at the high symmetry point K . Their existence, albeit not their position, is protected by the mechanism described by Zak [18] , relying upon a combination of symmetry and continuity of the wave function. Basically, the matrix element between the two bands in question is not zero any more for k z >0 along Γ– K , nor is it along Γ– M , but it cannot be continuosly transformed from one line to the other without passing through zero at some point in between. For a detailed discussion we refer the reader to ref. 18 . As a result, the Dirac points form a 3D line meandering about the vertical line passing through the hexagonal K point (see Supplementary Fig. 1 ), which, if averaged over k z , projects onto this point. Note that this apparent deviation from the hexagonal symmetry is related to the ABC stacking pattern of the kagome layers. A downfolding into the hexagonal Brillouin zone results in a three-sheet Fermi surface with hexagonal symmetry. When doped, the Fermi surface consists of six tubes that slightly twist as we move along k z ( Fig. 2f,g ). Normal-state instabilities Next we want to check the system against normal-state electronic instabilities. In a strongly correlated system this cannot be adequately addressed within the DFT. Therefore, we have constructed a many-body model Hamiltonian that captures the most important interactions: where the first term is the effective Cu tight-binding Hamiltonian derived from the DFT band structure (see Methods). The onsite U and nearest-neighbour Coulomb repulsion V were estimated (see Supplementary Note 2 ) to be U=5-7eV and V=0.11eV. It is worth noting that the latter number is unexpectedly small. The reason for that is twofold: first, even at the exact n =4/3 filling, where the metallic density of states (DOS) is zero, the behaviour of the dielectric constant is nearly metallic at the relevant distances, albeit the asymptotic long-range behaviour is semiconducting, and the Coulomb interaction is well screened; second, even though the electronic structure is quasi-2D, it is by far not the same as an isolated plane as in graphene—each plane participates in screening interactions not only within the plane but also in all other planes. Mott–Hubbard instability ZnCu 3 (OH) 6 Cl 2 is a Mott insulator since the Cu state is half-filled and electron hopping incurs an energy cost of U . This is not the case in GaCu 3 (OH) 6 Cl 2 . Its filling of n =4/3 corresponds to one electron per site plus one extra electron per three sites. Suppose U =∞. Then exactly 1/3 of all sites are double, and the rest are single occupied. Thus, one electron per site will be localized and 1/3 of an electron mobile, and this mobility will not be impeded at all. This simplistic treatment suggests that the system will be metallic. To verify this, we applied to the Hamiltonian (1) the dynamical cluster approximation (DCA) within the rotationally invariant slave-boson (DCA(RISB)) formalism [19] , [20] in the saddle-point approximation (see Methods). As a minimal cluster we considered three sites. 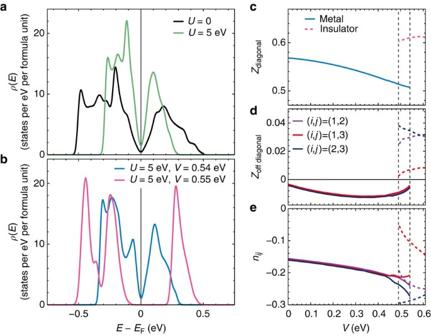Figure 4: Dynamical cluster approximation-like rotationally invariant slave boson results for GaCu3(OH)6Cl2. (a,b) Quasi-particle (QP) spectral function for different interactions on the three-site cluster. The curves are scaled with the respective onsite QP weightZ. (c–e) Cluster quantities with intersiteV: onsite QP weight (c), intersite QP weight (d), and intersite terms of the cluster orbital density matrix (e). Figure 4 shows our DCA(RISB) results in the paramagnetic regime. For U =5 eV, we observe a band narrowing, but the essential low-energy features, especially the pseudogap reflecting the Dirac points, remain. Thus, the onsite repulsion alone is insufficient to drive the system insulating at n =4/3. This is a key result, and we have confirmed it by using the more accurate continuous-time quantum Monte Carlo approach (see Supplementary Note 3 ). Figure 4: Dynamical cluster approximation-like rotationally invariant slave boson results for GaCu 3 (OH) 6 Cl 2 . ( a , b ) Quasi-particle (QP) spectral function for different interactions on the three-site cluster. The curves are scaled with the respective onsite QP weight Z . ( c – e ) Cluster quantities with intersite V : onsite QP weight ( c ), intersite QP weight ( d ), and intersite terms of the cluster orbital density matrix ( e ). Full size image Charge ordering Having verified the absence of a Mott–Hubbard transition, we turn to possible charge ordering, which in the limit U >> t is controlled by the intersite Coulomb repulsion V . At the mean-field level, the competition is between the energy gain of charge ordering, and the loss of kinetic energy. The former can be estimated from the fact that in the charge-ordered state no neighbouring sites are doubly occupied; thus, the nearest-neighbour repulsion is completely avoided. On the other hand, if all electrons are randomly distributed over all sites, each nearest-neighbour bond has (1/3) 2 =1/9 probability to have double occupancy on both sides, losing V /9 per bond, or 2 V /9 per site. The kinetic energy loss can be estimated as (2/3−1/6)=1/2 of the energy E 0 of non-interacting electrons on the kagome lattice ( E 0 ≈− t per site for n =4/3). (In the charge-disordered state any electron has a 2/3 probability that a given neighbouring site is single occupied and allows hopping, while in the ordered state half of the electrons are immobile, and the mobile ones have only 1/3 of the nearest neighbours single occupied.) Comparing 2 V /9 and 0.5 t we conclude that the system may develop charge ordering at V ≳ 2 t. Our DFT calculations yield t ~0.3 eV; however, one may expect a renormalization due to correlation effects; a factor of 2 is reasonable for Cu d electrons t ren ~ t /2 and we get V c ~2 t ren ~0.3 eV. This value is much larger than the V estimated for GaCu 3 (OH) 6 Cl 2 , and, therefore, it should remain a uniform metal. Again, we subjected these qualitative arguments to a numerical test, solving equation (1) within the DCA(RISB) for U =5 eV and different V values. At a critical V c =0.54 eV ( Fig. 4b,c ), well above the estimated value of V (≈0.11 eV), the system charge orders and loses its metallicity, consistent with the qualitative arguments above. Interestingly, close to and inside the insulating phase the system shows substantially increased values of the intersite terms in the quasi-particle weight ( Fig. 4d ) as well as in the cluster orbital density matrix ( Fig. 4e ). Inspection of the slave-boson multiplet amplitudes reveal an insulator composed of dominant coherent superpositions of the four-particle triangular cluster states with one double-occupied site and two single-occupied sites with different spin orientation, a reflection of proximity to charge ordering at V c =0.54 eV. Note that in our functional renormalization group (fRG) calculations, described below, the problem of the phase instabilities is approached from the opposite limit, namely the itinerant/weak coupling limit, valid at U ≲ t , appropriate for addressing the superconductivity. It is worth mentioning though, that in fRG the V c needed to stabilize the leading charge-ordering instability was also far greater than the realistic range of V . Ferromagnetism We consider next the possibility of a ferromagnetic instability. It is well known that Hubbard models with very large U / t and away from half-filling show a propensity for so-called Nagaoka ferromagnetism [21] . Existing calculations [22] suggest that GaCu 3 (OH) 6 Cl 2 is far from the Nagaoka regime. However, these works did not consider states with partial spin polarization, which are natural in a metallic system. Let us first estimate the effective magnetic interactions at the mean-field level by comparing the superexchange J ex ~4 t 2 / U ~70 meV and the ferromagnetic kinetic energy gain per bond, times the number of mobile electrons per site ( E KE = E 0 /3 × 1/3~30 meV). E KE < J ex , suggesting a spin liquid without a long range order. However, this estimate also does not account for partial polarization, and in fact shows that the two competing interactions are of the same order of magnitude. Therefore we looked for ferromagnetism with the DCA(RISB), and found no ferromagnetism at n =4/3 (Dirac metal) and n ≲ 4/3 (hole doping) for any reasonable parameters. In contrast, with electron doping ( n >4/3), as the superexchange is gradually suppressed, ferromagnetism becomes increasingly more favourable. The importance of electron itinerancy is particularly clear from our weak coupling fRG calculations (see Supplementary Note 4 ). By construction, fRG shows no instabilities for zero DOS, but as we dope away from the Dirac point (either holes or electrons) we find, at sufficiently large U , a ferromagnetic instability. It should be noted that fRG depends on resummation of all parquet diagrams, an approximation not rigorously justified when U exceeds the band width. As we do not see a clean divergent RG flow for the ferromagnetic channel, we cannot distinguish ferromagnetic fluctuations from a partially polarized ferromagnet. From the combined view of different methodologies, however, we can ascertain that the system is very close to a ferromagnetic instability; whether it is realized in GaCu 3 (OH) 6 Cl 2 , we cannot be sure. But, importantly, strong ferromagnetic fluctuations are essential for unconventional superconductivity, as discussed in the next section. Superconductivity Finally, we investigate the possibility of superconductivity in GaCu 3 (OH) 6 Cl 2 . Obviously, when the Fermi level is exactly at the Dirac point the effective DOS (averaged over the cutoff energy) is small, of the order of , where the cutoff is set at the exchange energy J ex ; υ F is the Dirac velocity and a is the lattice parameter. (Not only is the coupling constant λ small in this case, one should also keep in mind that when N (0)=0, and only N eff ≠0, the critical temperature [23] T c ∝ exp(−1/ λ 2 ) rather than exp(−1/ λ ).) However, if the Ga substitution is incomplete and the Fermi surfaces form narrow cylinders ( Fig. 2f,g ) one expects sizeable coupling with spin excitations. In a semiclassical picture, when an antiferromagnetic ground state is assumed, the relevant excitations are acoustic paramagnons (see ref. 24 ). Such acoustic (that is, soft at q →0, whether they correspond to ferro- or antiferromagnetic correlations inside the unit cell) paramagnons should lead to an f -wave superconductivity; indeed, in a hexagonal Brillouin zone the six K-points related by the rotational symmetry ( Supplementary Fig. 1 ) can be separated into two subsets, K and K ′, such that all points of a given subset are also connected by translational symmetry. Given that the superconducting order parameter has to honour translational symmetry (but not necessarily the rotational one), we see that as we go around the Brillouin zone the phase factors between the consecutive pockets (neglecting intrapocket variations) vary as φ , φ′ , φ , φ′ , φ , φ ′, corresponding to an L =3 ( f -wave) harmonic. Indeed there exists a state [25] , often labelled B 1 u , with the order parameter transforming as so that φ =− φ ′. In this case the intrapocket (for example, small q ) interaction is attractive and pairing, while the interpocket one is repulsive and pairbreaking. However, the interpocket interaction is suppressed (assuming an acoustic spectrum) as ( k F / G ) 2 , with the distance G = K – K ′. One can estimate the BCS T c = ω exp(−1/ λ ), where ω ~ Jk F a (ref. 24 , equation (2.23)), and λ ~ t 2 N ( E F )/ ω ~ t/J. We see that the coupling constant is roughly independent of doping, the prefactor changes approximately as a square root of doping and one can expect a sizeable T c for k F ≲ G /2 (the maximum possible value before changing the topology). For λ ~1, which seems to be a conservative estimate, and k F ~ G /4 we get T c ~0.07 J ~30 K for J ~40 meV. Note that in this regime dependence on λ is close to linear. Taking λ /2 raises the estimate for T c to 60 K. Note that such an analysis is not anymore that straightforward when one considers a realistic spin-disordered ground state since the magnetic fluctuation spectrum becomes more complex ( cf ., for example, ref. 26 ). All these estimates are orders of magnitude at best, therefore we turn again to a quantitative treatment in terms of multi-sublattice fRG [27] , [28] . Since superconductivity is an itinerant effect, the inherent fRG assumption of weak coupling should be acceptable. Around n =4/3 and constraining ourselves to the superconducting channel, which, from a Kohn–Luttinger perspective, would become the leading channel for sufficiently weak interactions, we find a clear preference for nodeless f -wave superconductivity, as anticipated from the qualitative argument above. The calculated gaps, while changing sign between the pockets, remain uniform inside each pocket (see Supplementary Fig. 3 ). It is worth noting that the disorder introduced by Zn doping, while weak, might even, counterintuitively, support superconductivity in this limit [29] . Finally, a subtlety could arise for significant V : In order to avoid onsite and nearest-neighbour repulsion, this could drive a transition from a nodeless B 1 u f -wave to a nodal B 2 u f -wave [30] , but for realistic values of V this is highly unlikely. Conclusions This work opens many interesting avenues towards novel physics in electron-doped herbertsmithite compounds. Bridging between an RVB scenario of frustrated magnetism for x =0 and a correlated Dirac metal at x =1, Zn 1− x Ga x Cu 3 (OH) 6 Cl 2 promises to exhibit a plethora of unconventional electronic phases as a function of doping, temperature and disorder as discussed in the previous sections. Even if a solid solution 0< x <1 (which would be an ultimate bonanza of novel physics) would not be realized experimentally, pure GaCu 3 (OH) 6 Cl 2 ( x =1) and its slightly hole doped version ( x ≲ 1) should be highly interesting systems. According to our analysis, in this regime (close to the Dirac points) the two leading candidates for the low-temperature ground state are weak ferromagnetism and f -wave superconductivity. Further experimental and theory work shall decide who the winner is in their competition. First-principles calculations For structural optimization and to probe structural stability we used the projector augmented wave method as implemented in the VASP package [31] , [32] , with the generalized gradient approximation (GGA) functional [33] . For the calculation of the dielectric constant (see Supplementary Note 2 ) we used the linear augmented plane wave method as implemented in the WIEN2k package [34] . Electronic structure plots of GaCu 3 (OH) 6 Cl 2 , presented in this work, as well as the tight-binding parameters, were obtained using the full-potential local orbital (FPLO) package [35] together with the GGA [33] functional. For the DOS in Fig. 2d , we use a very dense 100 × 100 × 100 k mesh. To obtain a tight-binding representation of the Cu bands near the Fermi level, we project the (Kohn–Sham) Bloch states onto localized orbitals using projective Wannier functions within the FPLO basis as described in ref. 36 . DCA(CT-QMC) We considered the DCA with N c =3 sites in combination with an interaction-expansion continuous-time quantum Monte Carlo approach as an exact impurity solver [37] in order to account for quantum as well as short-range spatial fluctuations beyond static mean-field theory. DCA(RISB) We applied DCA to the RISB formalism [19] , [20] in the saddle-point approximation. The kagome lattice calls for the minimal cluster of three sites, which was thus used for the calculations. Within the RISB scheme the electron’s quasiparticle character (fermionic f vσ ) and its high-energy excitations (taken into account by the set of slave bosons { φ }) are decomposed on the operator level through , where v is a generic orbital/site index and σ =↑, ↓. The electronic self-energy Σ( ω ) at the saddle point is local and incorporates terms linear in frequency ω , as well as static renormalization Σ stat , that is, Σ( ω )=(1− Z −1 ) ω +Σ stat , wherein Z is the usual quasiparticle weight matrix. For more details see ref. 20 . Note that the similarly formulated single-site approach is very similar to the multi-orbital Gutzwiller technique [38] . Functional renormalization group We employed multi-sublattice functional RG [27] , [28] to investigate the superconducting instability for a herbertsmithite Fermiology interpolating from the Zn limit at half filling to the hole-doped Ga limit. For the calculations we considered the effective two-dimensional band structure obtained from our ab initio calculations. How to cite this article: Mazin, I. I. et al. Theoretical prediction of a strongly correlated Dirac metal. Nat. Commun. 5:4261 doi: 10.1038/ncomms5261 (2014).